Cross-talk between KLF4 and STAT3 regulates axon regeneration Cytokine-induced activation of signal transducer and activator of transcription 3 (STAT3) promotes the regrowth of damaged axons in the adult central nervous system (CNS). Here we show that KLF4 physically interacts with STAT3 upon cytokine-induced phosphorylation of tyrosine 705 (Y705) on STAT3. This interaction suppresses STAT3-dependent gene expression by blocking its DNA-binding activity. The deletion of KLF4 in vivo induces axon regeneration of adult retinal ganglion cells (RGCs) via Janus kinase (JAK)–STAT3 signalling. This regeneration can be greatly enhanced by exogenous cytokine treatment, or removal of an endogenous JAK–STAT3 pathway inhibitor called suppressor of cytokine signalling 3 (SOCS3). These findings reveal an unexpected cross-talk between KLF4 and activated STAT3 in the regulation of axon regeneration that might have therapeutic implications in promoting repair of injured adult CNS. Although regrowth of damaged axons is crucial for neural repair, axons in the adult CNS fail to regenerate after injury. This failure is caused by the presence of inhibitory molecules and the absence of intrinsic regenerative capacity of mature neurons [1] , [2] , [3] . Removing these inhibitory influences can lead to limited axon growth in the adult CNS [4] , [5] , [6] . For example, regeneration of RGCs could be significantly enhanced by individual or combined deletion of phosphatase and tensin homologue (PTEN), a negative regulator of mammalian target of rapamycin, and SOCS3, a negative regulator of the JAK–STAT pathway [7] , [8] , [9] . Compared with the CNS, neurons in the peripheral nervous system exhibit a greater ability for regeneration and outgrowth after injury [10] . Cytokines such as interleukin 6 were found to be upregulated in axotomized dorsal root ganglion neurons and/or Schwann cells in the lesion sites, suggesting that cytokine-induced activation of the JAK–STAT pathway is involved in axon regeneration after injury [11] , [12] . Indeed, a rapid increase of signal transducer and activator of transcription 3 (STAT3) phosphorylation and nuclear translocation were found following peripheral facial nerve injury [13] . Activation of the JAK–STAT3 pathway also correlates with enhanced regenerative responses of dorsal root ganglion neurons [14] . Treatment with inhibitors for JAK–STAT3 abolishes the conditioning lesion-induced axon growth of the dorsal column [15] . In the eye, intraocular inflammation caused by a lens injury enhances neuronal survival and axonal regeneration of RGCs [16] . The inflammation-induced cytokine signalling, via proteins such as ciliary neurotrophic factor (CNTF) and leukaemia inhibitory factor (LIF), is critical for this process, as the lens injury-induced effects are reduced in Cntf −/− mice and completely lost in mice with combined deletion of Cntf and Lif [17] . Importantly, removing SOCS3, a feedback inhibitor of JAK–STAT signalling, can enhance axon growth in a STAT3-dependent manner [7] . Together, these data indicate that cytokine-induced JAK–STAT3 signalling has a positive role in the regulation of axon regeneration in both peripheral nervous system and CNS. We recently found that KLF4 modulates the JAK–STAT3 pathway in cortical neural progenitors [18] . KLF4, a zinc-finger-containing transcription factor, regulates skin barrier formation and differentiation of goblet cells in the colon during mouse development [19] , [20] . It is one of the original four factors that reprogram somatic cells to become induced pluripotent stem cells by direct interactions with OCT4 and SOX2 (refs 21 , 22 ). KLF4 is induced by STAT3, and both transcription factors have critical roles in maintaining self-renewal of embryonic stem cells [23] , [24] , [25] . In the CNS, KLF4 controls proliferation and differentiation of neural stem cells as well as radial neuronal migration [18] , [26] . Interestingly, KLF4 is also developmentally regulated in RGCs, and its deletion enhances axon regeneration, although the underlying mechanism is not clear [27] . In this study, we examined the cross-talk between KLF4 and JAK–STAT signalling. We found that KLF4 associates with and blocks the activity of phosphorylated STAT3 (pSTAT3). Importantly, the inhibitory function of KLF4 on STAT3 signalling contributes to the failure of injured RGCs to regenerate. KLF4 associates with pSTAT3 We performed co-immunoprecipitation experiments to examine a potential interaction between KLF4 and STAT3. FLAG-tagged KLF4 was precipitated from transfected COS7 cells and examined for binding of endogenous STAT3 by western blotting. Indeed, a slower migrating form of STAT3 was detected in the immunoprecipitates ( Fig. 1a ). As STAT3 is frequently phosphorylated by cytokine-induced signalling, we treated cells with LIF for 20 min before immunoprecipitation and found that KLF4 is specifically associated with the phosphorylated form of STAT3 (pSTAT3), which was detected with an antibody against phospho-Y705 ( Fig. 1b ). Subcellular fractionation further showed that KLF4 can bind to pSTAT3 in both the nucleus and the cytoplasm ( Supplementary Fig. S1 ). 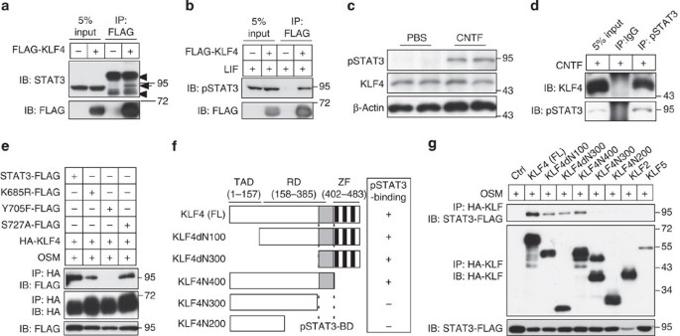Figure 1: KLF4 specifically associates with phosphorylated STAT3. (a) KLF4 associates with a modified form of STAT3 (indicated by an arrow) in COS7 cells. Arrow heads indicate non-specific protein bands. (b) KLF4 binds to phosphorylated STAT3 (pSTAT3) in COS7 cells treated with LIF. (c) CNTF treatment increases the endogenous level of pSTAT3 in mouse retinas. β-actin was used as a loading control. (d) Interaction of endogenous KLF4 and pSTAT3 in mouse retinas. IgG was used as a control. (e) Binding of KLF4 to STAT3 requires phosphorylation of Y705 but not other modifications on STAT3. (f) Diagram to show domain structure of full-length (FL) KLF4 and its truncation mutants. Their ability to bind to pSTAT3 is also indicated with either a ‘+’ (binding) or a ‘−’ (no binding). TAD, transactivation domain; RD, repression domain; ZF, zinc-fingers; pSTAT3-BD, pSTAT3-binding domain in KLF4. (g) Mapping pSTAT3-binding regions in KLF4 by co-immunoprecipitation. As controls, neither KLF2 nor KLF5 binds to STAT3. Molecular size markers are in kDa. Figure 1: KLF4 specifically associates with phosphorylated STAT3. ( a ) KLF4 associates with a modified form of STAT3 (indicated by an arrow) in COS7 cells. Arrow heads indicate non-specific protein bands. ( b ) KLF4 binds to phosphorylated STAT3 (pSTAT3) in COS7 cells treated with LIF. ( c ) CNTF treatment increases the endogenous level of pSTAT3 in mouse retinas. β-actin was used as a loading control. ( d ) Interaction of endogenous KLF4 and pSTAT3 in mouse retinas. IgG was used as a control. ( e ) Binding of KLF4 to STAT3 requires phosphorylation of Y705 but not other modifications on STAT3. ( f ) Diagram to show domain structure of full-length (FL) KLF4 and its truncation mutants. Their ability to bind to pSTAT3 is also indicated with either a ‘+’ (binding) or a ‘−’ (no binding). TAD, transactivation domain; RD, repression domain; ZF, zinc-fingers; pSTAT3-BD, pSTAT3-binding domain in KLF4. ( g ) Mapping pSTAT3-binding regions in KLF4 by co-immunoprecipitation. As controls, neither KLF2 nor KLF5 binds to STAT3. Molecular size markers are in kDa. Full size image To examine the interaction between endogenously expressed KLF4 and pSTAT3, we used mature RGCs as they are known to express a higher level of KLF4 (refs 27 , 28 ). As the level of pSTAT3 is low under normal conditions, we injected CNTF into the vitreous of adult mouse retinas to increase the level of pSTAT3 ( Fig. 1c ). Five hours later, pSTAT3 was immunoprecipitated from dissociated retinal cells. Consistently, endogenous KLF4 was specifically associated with pSTAT3 ( Fig. 1d ). Cytokines induce posttranslational modifications of STAT3, such as phosphorylation and acetylation. These modifications lead to an ‘activated’, dimerized form of STAT3 that functions as a transcriptional activator [29] . To determine which modification of STAT3 is required for its binding to KLF4, we cotransfected COS7 cells with HA-tagged KLF4 and various FLAG-tagged STAT3 mutants. These point mutations were designed to abolish either phosphorylation (Y705F and S727A) or acetylation (K685R) [29] . HA-tagged KLF4 was precipitated from whole-cell extracts following a 30-min pretreatment with oncostatin M (OSM), a pleiotropic IL6-like cytokine. Similar to wild-type STAT3, the S727A and K685R mutants strongly bind to KLF4 ( Fig. 1e ). In contrast, the Y705F mutant is no longer detected in the precipitates, indicating that phosphorylation at Y705 is critical for the interaction between STAT3 and KLF4. We mapped a region in KLF4 that is required for association with pSTAT3. Deletion of up to 300 amino acids (aa) from the amino terminus (KLF4dN100 and KLF4dN300) or removal of the zinc-fingers in the carboxyl terminus (KLF4N400) has no significant effect on KLF4 binding to pSTAT3 ( Fig. 1f,g ). In contrast, a mutant lacking 183 aa from the C terminus (KLF4N300) is no longer able to bind to pSTAT3, suggesting that the STAT3-binding domain in KLF4 is located in a region covering 301–400 aa ( Fig. 1f,g ). KLF4 inhibits cytokine-induced STAT3 activity We examined the effect of KLF4 on STAT3 signalling using a luciferase reporter (4 × M67 p TATA - TK - Luc ) containing four copies of consensus STAT3-binding sites [30] . Treatment of transfected COS7 cells with cytokine, OSM, induced robust activity of this reporter, which requires phosphorylation of Y705 but not acetylation of K685 of STAT3 ( Fig. 2a ). Interestingly, expression of the full-length KLF4 completely inhibited OSM-induced reporter activity. In contrast, truncation mutants of KLF4 (KLF4N200 and KLF4N300) that lack the ability to bind pSTAT3 were no longer able to block cytokine-induced reporter activity ( Fig. 2b ). To further confirm the inhibitory role of KLF4 on STAT3 activity, we used another luciferase reporter ( Sprr1a-Luc ) containing the promoter region of Sprr1a . Sprr1a has been proposed as a downstream target of the STAT3 signalling pathway [31] , and its proximal promoter region harbours a consensus STAT3-binding site. COS7 cells were cotransfected with Sprr1a-Luc and with plasmids expressing STAT3 and/or KLF4. Under basal conditions, the Sprr1a-Luc reporter exhibited only minimal activity even in the presence of exogenous wild-type STAT3 ( Fig. 2c ). OSM-treatment induced about a 15-fold increase of reporter activity. This required phosphorylation of Y705 of STAT3, as cytokine-induced activity was largely diminished when the STAT3-Y705F mutant was included. Once again, co-expression of KLF4 completely abolished OSM-induced Sprr1a-Luc activity ( Fig. 2c ). 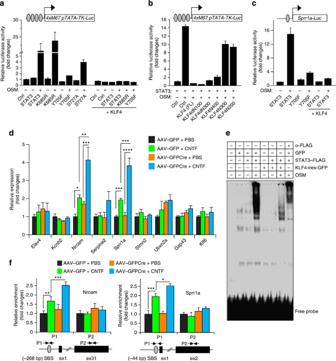Figure 2: KLF4 inhibits cytokine-induced STAT3 activity. (a,b) KLF4 suppresses the activity of a STAT3-dependent luciferase reporter in COS7 cells (means±s.e.m.;n=3). This reporter contains four copies of consensus STAT3-binding sites and requires cytokine-induced phosphorylation of Y705 for its activity (a). KLF4-truncation mutants that do not bind pSTAT3 lack the ability to suppress this reporter (b). Ctrl: cells transfected with an empty vector as controls. (c) KLF4 inhibits the OSM-induced and STAT3-dependent activity of a reporter from theSprr1agene (means±s.e.m.;n=3). (d) qRT-PCR analysis showing that KLF4 deletion enhances CNTF-induced gene expression in retinas ofKlf4f/fmice (means±s.e.m.;n=3; *P<0.04, **P<0.03, ***P<0.02, and ****P<0.001 by Student’st-test). (e) KLF4 disrupts DNA-binding activity of STAT3 detected by electrophoretic mobility shift assays. Nuclear extracts from GFP-transfected COS7 cells were used as controls. The inclusion of an antibody against FLAG-tagged STAT3 leads to a supershift, indicating STAT3-dependent DNA-binding activity. (f) ChIP assays showing that KLF4 deletion enhances CNTF-induced pSTAT3-binding to its target genes in retinas ofKlf4f/fmice (means±s.e.m.;n=3; *P<0.04, **P<0.03, and ***P<0.02 by Student’st-test). The positions of primers (P1 or P2) used for qPCR are indicated. ex, exon; SBS, STAT3-binding site. Figure 2: KLF4 inhibits cytokine-induced STAT3 activity. ( a , b ) KLF4 suppresses the activity of a STAT3-dependent luciferase reporter in COS7 cells (means±s.e.m. ; n =3). This reporter contains four copies of consensus STAT3-binding sites and requires cytokine-induced phosphorylation of Y705 for its activity ( a ). KLF4-truncation mutants that do not bind pSTAT3 lack the ability to suppress this reporter ( b ). Ctrl: cells transfected with an empty vector as controls. ( c ) KLF4 inhibits the OSM-induced and STAT3-dependent activity of a reporter from the Sprr1a gene (means±s.e.m. ; n =3). ( d ) qRT-PCR analysis showing that KLF4 deletion enhances CNTF-induced gene expression in retinas of Klf4 f/f mice (means±s.e.m. ; n =3; * P <0.04, ** P <0.03, *** P <0.02, and **** P <0.001 by Student’s t -test). ( e ) KLF4 disrupts DNA-binding activity of STAT3 detected by electrophoretic mobility shift assays. Nuclear extracts from GFP-transfected COS7 cells were used as controls. The inclusion of an antibody against FLAG-tagged STAT3 leads to a supershift, indicating STAT3-dependent DNA-binding activity. ( f ) ChIP assays showing that KLF4 deletion enhances CNTF-induced pSTAT3-binding to its target genes in retinas of Klf4 f/f mice (means±s.e.m. ; n =3; * P <0.04, ** P <0.03, and *** P <0.02 by Student’s t -test). The positions of primers (P1 or P2) used for qPCR are indicated. ex, exon; SBS, STAT3-binding site. Full size image Next, we analysed the role of KLF4 on the expression of endogenous STAT3-responsive genes in mouse retinas. KLF4 was deleted by intravitreal injection of adeno-associated virus (AAV) expressing green fluorescent protein (GFP) and Cre fusion protein (AAV–GFPCre) into mice harbouring floxed alleles of Klf4 ( Klf4 f/f ). AAV expressing GFP alone (AAV–GFP) was used as a control. Both GFP and GFPCre were under the regulation of human synapsin I promoter to specifically target neurons. Immunohistochemistry analysis showed that more than 80% of RGCs in the adult mouse retina could be targeted by injected AAV ( Supplementary Fig. S2 ). Two weeks post AAV injection, CNTF was intravitreally applied for 24 h to activate endogenous STAT3. Mice injected with PBS were used as controls. Western blot analysis showed that deletion of KLF4 did not change the expression of either pSTAT3 or total STAT3 ( Supplementary Fig. S3 ). Based on microarray analysis [9] , nine genes were chosen as candidate downstream targets of STAT3. Among these, the expression of Nrcam and Sprr1a was significantly induced by CNTF treatment ( Fig. 2d ). Importantly, deletion of KLF4 further greatly enhanced the expression of these two genes, indicating that endogenous KLF4 normally suppresses their response to cytokine-induced signalling. To tease out the mechanism by which KLF4 inhibits STAT3 signalling, we examined the effect of KLF4 on the DNA-binding activity of STAT3 by electrophoretic mobility shift assay. Electrophoretic mobility shift assay was performed using an oligonucleotide probe containing two consensus STAT3-binding sites and nuclear extracts from COS7 cells. Without cytokine treatment, neither STAT3 nor KLF4 had any effect on probe mobility. In contrast, treatment with OSM induced a large shift on probe mobility. This shift was dependent on activated STAT3, as it could be super shifted with an antibody against the epitope tag on STAT3. Remarkably, co-expression of KLF4 largely abolished the cytokine-induced DNA-binding activity of STAT3 ( Fig. 2e ). We then used chromatin immunoprecipitation assays to determine the effect of KLF4 on the binding of pSTAT3 to its target genes. Endogenous KLF4 was removed by intravitreal injection of AAV–GFPCre into the retinas of Klf4 f/f mice. Klf4 f/f mice injected with AAV–GFP were used as controls. Two weeks post AAV injection, endogenous STAT3 was activated by intravitreal injection of CNTF. Genomic DNA bound by activated STAT3 was immunoprecipitated with an antibody specific for pSTAT3 and was then quantified by qPCR. Treatment with CNTF induced significant binding of pSTAT3 to the proximal promoter region of the Nrcam or Sprr1a gene that harbours a consensus STAT3-binding site ( Fig. 2f ). Interestingly, deletion of KLF4 further enhanced binding of pSTAT3 to these sites. As controls, neither CNTF treatment nor deletion of KLF4 had any effect on the binding of pSTAT3 to the exon region of either Nrcam or Sprr1a gene that does not contain a STAT3-binding site ( Fig. 2f ). Together, these data indicate that KLF4 normally inhibits activated STAT3-dependent signalling by blocking its DNA-binding activity in the nucleus. KLF4 regulates axon regeneration through JAK–STAT3 signalling We used the optic nerve crush model to examine the biological function of this KLF4–pSTAT3 interaction, as both KLF4 and STAT3 signalling have been separately implicated in the regulation of axonal regeneration of injured RGCs [7] , [27] . Although knocking out KLF4 during development enhances axonal growth of adult RGCs [27] , it is not clear whether acute deletion of KLF4 in adulthood has a similar effect. We performed intravitreal injection of AAV–GFPCre to remove endogenous KLF4 in adult Klf4 f/f mice. AAV–GFP was used as a control. Two weeks after intravitreal AAV injection, mice were subjected to optic nerve crush ( Fig. 3a ). Two more weeks later, Alexa fluor 594-conjugated cholera toxin beta subunit (CTB), an anterograde tracer, was injected intravitreally to label RGC axons. Consistent with previous results [27] , acute deletion of Klf4 led to significant axonal regeneration of damaged RGCs ( Fig. 3b,c ). On the other hand, Klf4 deletion had no effect on RGC survival, indicated by a similar number of surviving TUJ1 + RGCs in the retinas injected with AAV–GFPCre and control AAV–GFP ( Supplementary Fig. S4 ). 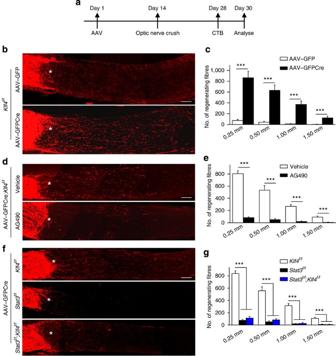Figure 3: KLF4 regulates axon regeneration through JAK–STAT3 signalling. (a) Experimental scheme. CTB, cholera toxin beta subunit. (b,c) Acute deletion ofKlf4leads to enhanced axon growth after optic nerve crush. Axons were traced with CTB that was injected into the vitreous and estimated at the indicated distance distal to the crush sites (means±s.e.m.;n=3 and 5 for AAV-GFP and AAV–GFPCre groups, respectively; ***P<0.001 by ANOVA with Bonferroni’sposthoctest). (d,e) Treatment with AG490, an inhibitor of JAK-STAT signalling, diminishesKlf4deletion-induced axon growth (means±s.e.m.;n=4 and 5 for vehicle and AG490 groups, respectively; ***P<0.001 by ANOVA with Bonferroni’spost hoctest). (f,g) Removal ofStat3completely abolishes axon regeneration induced byKlf4deletion (means±s.e.m.;n=3, 3, and 5 forKlf4f/f,Stat3f/f, andStat3f/f;Klf4f/fmice, respectively; ***P<0.001 by ANOVA with Bonferroni’spost hoctest). Asterisks, crush sites; scales, 100 μm. Figure 3: KLF4 regulates axon regeneration through JAK–STAT3 signalling. ( a ) Experimental scheme. CTB, cholera toxin beta subunit. ( b , c ) Acute deletion of Klf4 leads to enhanced axon growth after optic nerve crush. Axons were traced with CTB that was injected into the vitreous and estimated at the indicated distance distal to the crush sites (means±s.e.m. ; n =3 and 5 for AAV-GFP and AAV–GFPCre groups, respectively; *** P <0.001 by ANOVA with Bonferroni’s post hoc test). ( d , e ) Treatment with AG490, an inhibitor of JAK-STAT signalling, diminishes Klf4 deletion-induced axon growth (means±s.e.m. ; n =4 and 5 for vehicle and AG490 groups, respectively; *** P <0.001 by ANOVA with Bonferroni’s post hoc test). ( f , g ) Removal of Stat3 completely abolishes axon regeneration induced by Klf4 deletion (means±s.e.m. ; n =3, 3, and 5 for Klf4 f/f , Stat3 f/f , and Stat3 f/f ;Klf4 f/f mice, respectively; *** P <0.001 by ANOVA with Bonferroni’s post hoc test). Asterisks, crush sites; scales, 100 μm. Full size image Our finding that KLF4 inhibits activated STAT3 suggests that the enhanced regeneration observed in Klf4 -deleted retina ( Klf4 f/f with AAV–GFPCre) might be due to releasing the inhibitory effect of KLF4 on STAT3. We tested this hypothesis by employing both pharmacological and genetic approaches. First, we used a JAK inhibitor, AG490, to block activation of STAT3 (refs 32 , 33 , 34 ). Two weeks post injection of AAV–GFPCre, AG490 was applied twice into the intravitreal space of Klf4 f/f retina: once immediately after nerve crush and once at 3 days later. Vehicle treatments were used as controls. Although AG490 had no major effect on RGC survival ( Supplementary Fig. S5 ), it caused a more than 15-fold reduction in regenerating axons at 1.5 mm distal to the crush site in Klf4 -deleted retinas ( Fig. 3d,e ). Second, we generated mutant mice carrying different alleles of Klf4 f/f and Stat3 f/f . The retinas of adult Klf4 f/f , Stat3 f/f and Klf4 f/f ; Stat3 f/f mice were unilaterally injected with AAV–GFPCre virus into the intravitreal space, followed by optic nerve crush at day 14, CTB injection at day 28, and analysis at day 30. Consistent with a previous report [9] , RGC axons of Stat3 -deleted mice do not regenerate. Importantly, double deletion of Stat3 and Klf4 completely abolished axonal regrowth of injured RGCs that was observed in the Klf4 -deleted retinas ( Fig. 3f,g ). Together, these data showed that Klf4 deletion-induced axonal regeneration requires JAK–STAT3 activity. Removal of SOCS3 enhances axon regeneration The above data demonstrates that KLF4 is an endogenous inhibitor of activated STAT3. Another endogenous inhibitor of the JAK–STAT pathway is SOCS3, which is induced by activated STAT3 as a feedback mechanism to restrict JAK activity [35] . As these two inhibitors regulate STAT3 activity through different mechanisms, we reasoned that axon growth could be enhanced by simultaneously removing these two inhibitors. AAV–GFPCre virus was intravitreally injected into the eyes of WT, Socs3 f/f or Klf4 f/f /Socs3 f/f mice. Sixteen days post nerve crush, Socs3 -deleted mice showed a significant increase in axon growth and survival of damaged RGCs when compared with their WT controls ( Fig. 4a–c ). Consistently, additional deletion of Klf4 had an additive effect on the number of regenerating axons, with threefold more axons at 1.5 mm distal to the injury site when compared with mice with the Socs3 deletion only. On the other hand, Klf4 deletion had no additional effect on the survival of injured RGCs ( Fig. 4a–c and Supplementary Fig. S6 ). 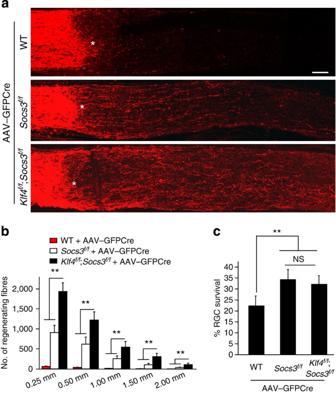Figure 4: Enhanced axon growth by co-deletion ofKlf4andSocs3. (a) Representative confocal images showing CTB-labelled axon fibres in mouse retinas with the indicated genotypes. Asterisks, crush sites; scale, 100 μm. (b) Estimated axon numbers at the indicated distance distal to the crush sites (means±s.e.m.;n=5; **P<0.01 by ANOVA with Bonferroni’spost hoctest). (c) Survival of TUJ1+RGCs 16 days post injury. The number of TUJ1+RGCs in the injured retina was normalized to that in the uninjured retina within the same animal (means±s.e.m.;n=5; **P<0.01 by ANOVA withpost hocTukey’s test; NS, not significant). Figure 4: Enhanced axon growth by co-deletion of Klf4 and Socs3 . ( a ) Representative confocal images showing CTB-labelled axon fibres in mouse retinas with the indicated genotypes. Asterisks, crush sites; scale, 100 μm. ( b ) Estimated axon numbers at the indicated distance distal to the crush sites (means±s.e.m. ; n =5; ** P <0.01 by ANOVA with Bonferroni’s post hoc test). ( c ) Survival of TUJ1 + RGCs 16 days post injury. The number of TUJ1 + RGCs in the injured retina was normalized to that in the uninjured retina within the same animal (means±s.e.m. ; n =5; ** P <0.01 by ANOVA with post hoc Tukey’s test; NS, not significant). Full size image KLF4 deletion enhances cytokine-induced axon repair While it was significant when compared with AAV–GFP-injected controls, axon growth in AAV–GFPCre-injected Klf4 f/f RGCs was modest ( Fig. 3a,d ). This could be due to low levels of activated STAT3 in injured RGCs. Indeed, consistent with previously published results [7] , pSTAT3 was hardly detectable by immunohistochemistry in nerve-crushed retinas. To boost JAK–STAT signalling, we intravitreally injected CNTF to Klf4 f/f mice immediately after optic nerve crush and 3 days later. Compared with PBS-treated and AAV–GFP-injected control mice, CNTF treatment only produced a very limited increase in axon growth of injured RGCs ( Fig. 5a,b ). This could be as a result of strong inhibition conferred by endogenous KLF4 to pSTAT3. Supporting this hypothesis, we observed a dramatic enhancement of axon growth in CNTF-treated and AAV–GFPCre-injected Klf4 f/f retinas. KLF4-deletion led to a nearly 10-fold increase in the number of regenerating fibres at 1.5 mm distal to the crushed site compared with CNTF-treated control (AAV–GFP-injected) RGCs ( Fig. 5a,b ). Interestingly, a combination of KLF4 deletion and CNTF treatment (but neither alone) also resulted in a significant increase in the survival of injured RGCs ( Fig. 5c ). Together, these data indicate that growth and survival of injured axons could be dramatically promoted through a synergism induced by enhanced cytokine signalling and the removal of endogenous inhibitors. 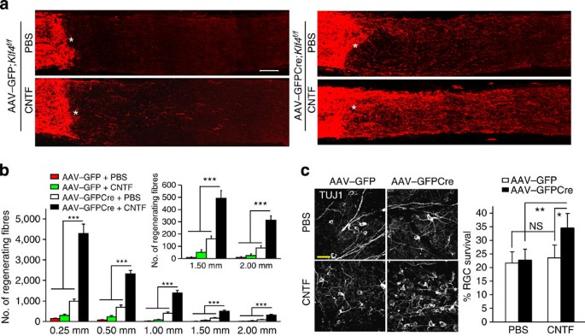Figure 5:Klf4deletion enhances cytokine-induced axon repair and survival. (a) Representative confocal images showing CTB-traced RGC axons 16 days post nerve crush. Asterisks, crush sites; scale, 100 μm. (b) Estimated axon numbers at the indicated distance to the crush sites (means±s.e.m.;n=5; ***P<0.001 by ANOVA with Bonferroni’spost hoctest). (c) Survival of TUJ1+RGCs 16 days post injury. Confocal images of TUJ+RGCs are shown in the left panels. The number of TUJ1+RGCs in the injured retina was normalized to that in the uninjured retina within the same animal (means±s.e.m.;n=5; *P<0.003 and **P<0.001 by ANOVA withpost hocTukey’s test; NS, not significant). Figure 5: Klf4 deletion enhances cytokine-induced axon repair and survival. ( a ) Representative confocal images showing CTB-traced RGC axons 16 days post nerve crush. Asterisks, crush sites; scale, 100 μm. ( b ) Estimated axon numbers at the indicated distance to the crush sites (means±s.e.m. ; n =5; *** P <0.001 by ANOVA with Bonferroni’s post hoc test). ( c ) Survival of TUJ1 + RGCs 16 days post injury. Confocal images of TUJ + RGCs are shown in the left panels. The number of TUJ1 + RGCs in the injured retina was normalized to that in the uninjured retina within the same animal (means±s.e.m. ; n =5; * P <0.003 and ** P <0.001 by ANOVA with post hoc Tukey’s test; NS, not significant). Full size image Cytokine-induced JAK–STAT3 signalling has emerged as a positive regulator of injured axon regrowth [10] , [36] . The results of this study demonstrate that KLF4 acts as an intrinsic inhibitor of this signalling pathway to suppress regeneration of injured RGC axons. Removing KLF4-mediated inhibition synergizes with cytokine signalling to greatly promote regeneration and survival of injured RGCs. In response to cytokines binding to their receptors on the cell surface, STAT3 is phosphorylated on Y705 by activated JAKs. This phosphorylation leads to dimerization and nuclear accumulation of STAT3, which then recognizes target DNAs and activates gene expression. Furthermore, STAT3 activity is regulated by the association with multiple cofactors. For example, a direct interaction with C-Jun or CBP/p300 promotes STAT3 activity, whereas binding of PIAS3 or Cyclin D1 represses its function [37] , [38] , [39] , [40] . Interestingly, the association of PIAS3 with STAT3 is detectable only in cells treated with cytokine [39] . SOCS3, a direct downstream target of activated STAT3, also restricts JAK–STAT signalling as a feedback mechanism [35] . Adding to this complex regulation of the JAK–STAT pathway is our current finding that KLF4 binds to and inhibits activated STAT3. Remarkably, the association of KLF4 with STAT3 specifically requires cytokine-induced phosphorylation of Y705. KLF4 is emerging as a key player in the regulation of multiple physiological and pathological processes in a cellular context-dependent manner. For example, KLF4 promotes maintenance of embryonic stem cells [41] and cellular reprogramming to pluripotency [42] , whereas it is also required for skin development and differentiation of colonic goblet cells [19] , [20] . KLF4 can function as either a tumour suppressor or an oncogene depending on tissue types [43] . Contrary to its positive role in embryonic stem cells and induced pluripotent stem cells, increased expression of KLF4 reduces self-renewal of neural stem cells and promotes their differentiation into glia-like cells [18] , [26] . A potential underlying mechanism by which KLF4 regulates neural stem cell behaviour is by enhancing JAK–STAT signalling [44] . In contrast, our current study demonstrates that suppressing activated STAT3 by KLF4 constitutes an intrinsic barrier for regeneration of damaged adult RGC axons. These data clearly indicate that the cellular milieu has an essential role in modulating KLF4-associated signalling and dictates its ultimate biological outputs. Inflammatory stimulation by lens injury or nerve crush induces expression of multiple cytokines, such as CNTF and LIF [16] , [17] , [45] , [46] . These cytokines, whether endogenously induced or further enhanced by exogenous treatment, promote axon growth after optic nerve injury [16] , [17] , [46] , [47] . However, the extent of axon regeneration under these conditions is modest [1] , [10] . This is very likely due to strong intrinsic inhibition on the cytokine-induced JAK–STAT signal transduction pathway. SOCS3, generally upregulated in axotomized RGCs following lens injury [48] , is such an intrinsic inhibitor, as its deletion significantly potentiates the effect of CNTF treatment on axon growth [7] . Similarly, results from this study demonstrate that KLF4 constitutes another strong inhibition of activated STAT3. Removal of this inhibition synergizes with cytokine signalling to greatly enhance the regenerative capacity and survival of damaged RGCs. Collectively, these data indicate that robust axon regeneration requires both positive inputs, such as cytokine-initiated signalling, and the removal of intrinsic barriers. As a potential therapeutic strategy for promoting survival and axon regrowth of damaged adult CNS neurons, a multipronged approach targeting several pathways might be essential. As previously demonstrated, co-deletion of PTEN and SOCS3 can initiate sustained axon regeneration [9] . A similar effect is expected by combining KLF4 deletion with other pathways, such as inhibition of PTEN or activation of mammalian target of rapamycin. A question is how to target KLF4, a transcription factor, for potential therapeutics. A strategy might be to develop small molecules to disrupt the interaction of KLF4 with pSTAT3. As endogenous KLF4 is a target of several microRNAs [49] , [50] , boosting expression of these microRNAs or exogenous delivery of miRNA mimics might also be practical alternatives. Animals The generation of Klf4 f/f , Socs3 f/f and Stat3 f/f mice has been previously described [19] , [51] , [52] . Unless otherwise indicated, mice with ages between 4–8 weeks were used. No significant phenotypic differences were detected between male and female mice; thus, both genders were included in the analysis. No statistical method was used to predetermine the sample size. The experiments were age and gender controlled. Mice with failed surgical procedures were excluded from analysis. The investigators were not blinded to allocation of animals during experiments and outcome assessment. All mice were housed under a 12 h light–dark cycle and had ad libitum access to food and water in a controlled animal facility. Experimental protocols were approved by the Institutional Animal Care and Use Committee at the University of Texas Southwestern Medical Center. Plasmids cDNAs encoding full length or truncated mouse KLF4 were amplified by PCR and individually inserted into the pCMX vector with either a FLAG-tag or an HA-tag at the amino terminus. MYC-tagged wild-type STAT3 and its mutants (K685R, Y705F and S727A) were generous gifts of Y. Eugene Chin (Brown University). The genes encoding wild-type STAT3 and its mutants were also subcloned into pRc/CMV vector (Invitrogen) with a coding sequence for a FLAG-tag at their amino termini. To create the Sprr1a-Luc reporter, a genomic fragment covering −973 bp to +46 bp of the Sprr1a gene was amplified by PCR and subcloned into pGL4.23 vector (Promega). STAT3-dependent reporter, 4 X M67 p TATA - TK - Luc, which contains four copies of STAT3-binding sites was obtained from Addgene [30] . All plasmids were confirmed by restriction digestion and/or sequencing. Cell culture and transfection COS7 cells (ATCC) were cultured in DMEM (Invitrogen) containing 10% fetal bovine serum (Invitrogen) and were transfected with PolyJet reagent (SignaGen Laboratories). For immunoprecipitation, the cells were treated with either LIF (100 ng ml −1 ) for 20 min or OSM (10 ng ml −1 ) for 30 min before harvest as indicated. For reporter assays, COS7 cells (30,000 per well) were sub-cultured in 48-well plates. After 24 h, cells were cotransfected with a reporter plasmid and plasmids expressing KLF4, STAT3 or STAT3 mutants as indicated. CMV-LacZ (25 ng) was also included in each transfection as a control for transfection efficiency. The total plasmid amount was kept at 200 ng for each transfection by adding corresponding empty vectors. Luciferase reporter assays Thirty-six hours after transfection, cells were treated with OSM (10 ng ml −1 ) or vehicle for 5 h when indicated. Immediately following treatment, cells were lysed and assayed for luciferase activity using the Dual-Light system (Applied Biosystems). Luciferase values were then normalized to that of β-galactosidase activity. All luciferase reporter assays were done in triplicates for at least twice. Immunoprecipitation and western blotting Cells were homogenized with a lysis buffer containing 50 mM Tris-HCl (pH 7.5), 150 mM NaCl, 1 mM EDTA, 0.5% sodium deoxycholate, 1% NP-40, 50 mM NaF, 0.5 mM PMSF, 1 mM Na 3 VO 4 , protease and phosphatase inhibitor cocktail (Roche). Protein concentrations in the cell lysates were determined using Bradford assays. Cell lysates (500–800 μg) were then incubated with either 10 μl anti-FLAG (M2, Sigma) or 10 μl anti-HA (3F10, Roche) affinity matrix as indicated for 2 h at 4 °C, followed by extensive washing with lysis buffer. To detect interaction between endogenous KLF4 and pSTAT3, 1–2 μl CNTF (10 μg ml −1 , Sigma) was injected into the vitreous space to enhance the level of pSTAT3. Five hours later, retinas were harvested and homogenized with lysis buffer. Retinal lysates (300 μg each) were then incubated with protein G-conjugated Dynabeads (Invitrogen) and a rabbit anti-pSTAT3 polyclonal antibody for 2 h at 4 °C, followed by washing with lysis buffer. Protein samples were then separated by 10% SDS–PAGE and transferred onto (polyvinylidene difluoride) membranes (Millipore). The membranes were sequentially blotted with the corresponding primary and secondary antibodies and processed for enhanced chemiluminescence detection (Amersham). The following antibodies were used: pSTAT3 (phospho-Y705, rabbit 1:1,000, Cell Signaling), STAT3 (mouse, 1:1,000, Cell Signaling), FLAG (rabbit or mouse, 1:1,000, Sigma), HA (rabbit, 1:1,000, Santa Cruz), and KLF4 (goat, 1:800, R&D). Full scans of all western blots are supplied in Supplementary Figs S7 and S8 . Electrophoretic mobility shift assays Synthetic oligonucleotides (5′-GAC GGT TCC CGT AAA TGC ATC AGG TTC CCG TAA ATG-3′) containing two consensus STAT3-binding sites (5′-TTC CCG TAA-3′) were annealed and labelled with 32 P-dCTP as a probe. To obtain nuclear extracts, COS7 cells were transfected with HA–KLF4 and/or FLAG–STAT3 as indicated. Forty-eight hours later, cells were treated with OSM (10 ng ml −1 ) for 30 min and then lysed in hypotonic buffer containing 10 mM HEPES (pH 7.8), 10 mM KCl, 2 mM MgCl 2 , 0.1 mM EDTA, 0.5 mM DTT, 0.5% NP-40, protease and phosphatase inhibitors (Roche). After a 15-min incubation period on ice, the concentration of NP-40 was increased to 1%. Cell lysates were then vortexed for 10 s and centrifuged for 3 min at 3,000 g and 4 °C. The pellets were collected and resuspended in extraction buffer containing 50 mM HEPES (pH 7.8), 50 mM KCl, 300 mM NaCl, 0.1 mM EDTA, 0.5 mM DTT, protease and phosphatase inhibitors. After vigorous shaking for 30 min at 4 °C, nuclear extracts were collected following centrifugation at 15,000 g for 10 min. Protein concentrations were measured by Bradford assays. Nuclear extracts (5 μg) were then incubated with 32 P-dCTP-labelled probes (2 × 10 5 c.p.m.) in binding buffer containing 10 mM HEPES (pH 7.8), 50 mM KCl, 1 mM EDTA, 10% glycerol, 1 mM DTT and 50 μg ml −1 poly(dI:dC) for 20 min at RT. For antibody-mediated supershift assays, 1 μg anti-FLAG antibody (M2, Sigma) was added and incubated for an additional 15 min. The protein–DNA complexes were separated by 4% non-denaturing polyacrylamide gels and detected by autoradiography. Intravitreal injection AAV–GFP (AAV2/9.hSynapsin.EGFP.WPRE.bGH) and AAV–GFPCre (AAV2/9.hSynapsin.HI.GFPCre.WPRE.SV40) were purchased from the University of Pennsylvania Vector Core. Viral titres were 0.5 × 10 12 to 1.0 × 10 12 genome copies (GC) ml −1 . After anaesthetization of young adult mice (~6 weeks), a small incision just posterior to the pars plana of the left eye was made by using the tip of a sharp 30-gauge needle. An injection needle (33 gauge) connected to a 5 μl Hamilton syringe was carefully inserted through the incision to inject 1 μl of AAV–GFPCre or AAV–GFP. Care was taken to avoid damage to the lens during injection. Where indicated, CNTF, AG490, or vehicle was similarly injected. Quantitative RT–PCR Adult Klf4 f/f mice were intravitreally injected with AAV–GFP or AAV–GFPCre. Two weeks post viral injections, 1–2 μl PBS or CNTF (10 μg ml −1 in PBS, Sigma) was also injected into the vitreous space. Twenty four hours later, retinas were dissected out under a microscope. Total RNAs from each individual retina were extracted using TRIzol reagents (Invitrogen) and an RNeasy Mini Kit (Qiagen). cDNAs were synthesized from 0.25 μg of total RNAs by using random primers and a SuperScript III kit (Invitrogen). Gene expression was analysed through the SYBR Greener system (Invitrogen) on a 384-well ABI 7900HT thermocycler (Applied Biosystems). The PCR programme consisted 2 min at 50 °C and 10 min at 95 °C, followed by 40 cycles of 15 s at 95 °C and 60 s at 58 °C. Primer quality was examined through dissociation curves. Relative gene expression was determined by the ΔΔCt method (where Ct is the threshold cycle) after normalizing to the expression of Hprt . Primer sequences are listed in Supplementary Table S1 . Chromatin immunoprecipitation Chromatin immunoprecipitation experiments were performed using retinas from young adult Klf4 f/f mice (~6 weeks). Two weeks post intravitreal injections of AAV–GFP or AAV–GFPCre, 1–2 μl PBS or CNTF (10 μg ml −1 ) was injected into the vitreous space. Six hours later, retinas were dissected and cross-linked with 1% formaldehyde for 15 min at RT, followed by addition of 1/20 volume of 2.5 M glycine to stop the reaction. Samples were then subjected to sonication (10% duty cycle, output 3, 12 cycles of a 10-sec pulse and a 20-sec break by using Sonicator XL2020, Misonix) to obtain DNA fragments ranging from 150–500 bp. Sonicated chromatin (150 μg determined by OD260) was incubated with a pSTAT3-specific antibody (rabbit anti phospho-Y705, 1 μg, Cell Signaling) and Protein G-coupled Dynabeads (Roche). A rabbit IgG was used as a negative control. After extensive washes and elution, cross-links were reversed at 65 °C overnight. DNAs were then purified by phenol/chloroform extraction and ethanol precipitation and were analysed by qPCR using the primers listed in Supplementary Table S1 . Optic nerve crush Two weeks following intravitreal viral injection, the left intraorbital optic nerve was surgically exposed and crushed at 1 mm distal to the optic disc with a pair of 15-degree angled jeweler’s forceps (Dumont #5; Roboz) for 5 s. Great care was taken to avoid damages to the ophthalmic artery. After surgery, ophthalmic Tobrex ointment was applied to prevent infection. When indicated, 1 μl CNTF (10 μg ml −1 in PBS, PeproTech) or 1 μl AG490 (5 mM in 50% ethanol, Sigma) was intravitreally injected immediately following injury and at 3 days later. Anterograde labelling and quantification of RGC axons Following anaesthesia, 1 μl cholera toxin subunit B (CTB, 2.5 μg μl −1 , Molecular Probes) was injected into the vitreous with a Hamilton syringe. Two days later, mice were deeply anaesthetized and sequentially perfused transcardially with PBS and 4% PFA. Both eyes with the optic nerve segment still attached were dissected out, postfixed in 4% PFA for 2 h, washed in PBS and cryoprotected with 30% sucrose in PBS for 24 h at 4 °C. Longitudinal sections of optic nerves were cut at 10 μm thickness with a Cryostat (Leica) and mounted onto Superfrost Plus microscope slides (Fisher). Regenerating axons were quantified [8] , [16] . Briefly, the total number of regenerating fibres in each retina was estimated by counting CTB-labelled fibers at the indicated distances (0.25 mm, 0.50 mm, 1.00 mm, 1.50 mm) distal to the crush site. The cross-sectional width of the nerves was measured at the counting points to calculate the number of axons per mm of nerve width. This number was averaged from five sections per animal. Σ ad , the total number of axons extending distance d in a nerve with a radius of r , was estimated by summing over all sections having a thickness t (10 μm): Σ ad = πr 2 × [average axons mm −1 ]/ t . Immunohistochemistry and quantification of RGC survival Whole-mount retinas or coronal retinal sections (14-μm thickness) were permeabilized with blocking buffer (5% BSA/0.25% TX-100 in PBS) and incubated with anti-TUJ1 antibody (mouse, 1:2,000, Covance) in blocking buffer overnight at 4 °C. After washing with PBS, samples were subsequently incubated with Alexa fluor 594-conjugated secondary antibody (1:1,000, Molecular Probes). Nuclei were counterstained with Hoechst 33,342 (Hst). Fluorescent images were acquired on a Zeiss LSM510 META confocal system. Each whole-mount retina was randomly sampled for TUJ1-positive RGCs from 15–20 fields in the ganglionic cell layer. The average number of TUJ1-positive RGCs per field in the injured left eye was compared with that in the unoperated right eye from the same animal to determine the relative ratio of viable RGCs. Statistical analysis Data are expressed as means±s.d. Statistical analysis was performed by either analysis of variance with Bonferroni’s or Tukey’s post hoc test for multiple comparisons or a two-tailed unpaired Student’s t -test. A P value of <0.05 was considered significant. How to cite this article: Qin, S. et al. Cross-talk between KLF4 and STAT3 regulates axon regeneration. Nat. Commun. 4:2633 doi: 10.1038/ncomms3633 (2013).